Monoallelic expression and epigenetic inheritance sustained by aTrypanosoma bruceivariant surface glycoprotein exclusion complex 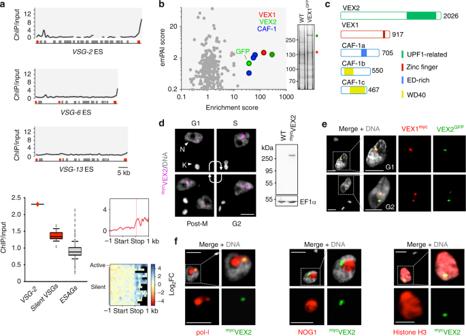Fig. 1 A subtelomere- andVSG-associated VEX-complex.aAffinity purification of VEX1myc-associated chromatin followed by sequencing (ChIP-seq). Enrichment traces over active (VSG-2) and silent (VSG-6,VSG-13)VSG-ESs with 1 kbp non-overlapping bins; red circles, promoters; red boxes,VSGs; grey boxes, expression-site associated genes (ESAGs). Box-plot depicting enrichment of the indicated CDSs. Centre lines show the medians; box limits indicate the 25th and 75th percentiles; whiskers extend from the 10th to the 90th percentile, outliers are shown. SilentVSGs,n= 18;ESAGs,n= 129. Metagene plot and the associated heat-map for active and silent telomericVSGs. The red bar on the metagene plot indicates the location of a highly conserved sequence in theVSG3’-untranslated region.bVEX1GFPimmunoprecipitation and proteomics. GFP-tag dependent enrichment from bloodstream formT. brucei. emPAI, exponentially modified protein abundance index. The inset shows immunoprecipitates and tag-dependent VEX1 (red) and VEX2 (green) bands highlighted in a silver-stained gel.cSchematic representation of VEX1 (Tb927.11.16920), VEX2 (Tb927.11.13380) and CAF-1 subunits (a, Tb927.8.3980; b, Tb927.10.7050; c, Tb927.11.4970) indicating conserved domains and motifs.dImmunofluorescence analysis during the cell cycle and protein-blot analysis ofmycVEX2 expression. N nucleus; K kinetoplast (mitochondrial genome).e,fImmunofluorescence-based colocalisation studies of VEX2GFPand VEX1myc(e) or a nucleolar (No) and ESB marker (pol-I, largest subunit), a nucleolar marker (NOG1) or Histone H3 (f). Ine, G1 or G2 cells are shown.d–fDNA was counter-stained with DAPI; the images correspond to maximal 3D projections of 0.1 μm stacks; scale bars 2 μm; the data are representative of independent biological replicates and independent experiments. Source data are provided as a Source Data file The largest gene families in eukaryotes are subject to allelic exclusion, but mechanisms underpinning single allele selection and inheritance remain unclear. Here, we describe a protein complex sustaining variant surface glycoprotein ( VSG ) allelic exclusion and antigenic variation in Trypanosoma brucei parasites. The VSG- exclusion-1 (VEX1) protein binds both telomeric VSG -associated chromatin and VEX2, an ortholog of nonsense-mediated-decay helicase, UPF1. VEX1 and VEX2 assemble in an RNA polymerase-I transcription-dependent manner and sustain the active, subtelomeric VSG -associated transcription compartment. VSG transcripts and VSG coats become highly heterogeneous when VEX proteins are depleted. Further, the DNA replication-associated chromatin assembly factor, CAF-1, binds to and specifically maintains VEX1 compartmentalisation following DNA replication. Thus, the VEX-complex controls VSG -exclusion, while CAF-1 sustains VEX-complex inheritance in association with the active- VSG . Notably, the VEX2-orthologue and CAF-1 in mammals are also implicated in exclusion and inheritance functions. In trypanosomes, these factors sustain a highly effective and paradigmatic immune evasion strategy. Antigenic variation and host immune evasion by parasites causing malaria [1] , giardiasis [2] and African trypanosomiasis [3] depend upon monoallelic and switchable variant surface antigen expression. Indeed, allelic exclusion governs the expression of many of the largest known gene-families, typically encoding cell-surface proteins in protozoa and mammals, and has major impacts on health and disease. In mammals, odour detection depends upon olfactory receptor exclusion [4] and B- and T-cell specificity depends upon immunoglobulin and surface receptor exclusion, respectively [5] . Selection of a single allele from a large gene family is thought to be inherently stochastic rather than deterministic and generates tremendous cellular diversity, upon which adaptive mechanisms operate. Notably, the diversity-generating exclusion systems of protozoan antigenic variation, and the host immune response, are mutually adaptive and in direct competition. Despite intense study, the molecular mechanisms facilitating the selection and maintenance of a single active allele, coordinated with heritable exclusion of all others, remain poorly understood. The African trypanosome, Trypanosoma brucei , is transmitted among mammalian hosts by tsetse-flies and, due to effective immune evasion, causes chronic and lethal infections, specifically sleeping-sickness in humans and nagana in cattle. In these parasites RNA polymerase-I (pol-I) transcribes a single, dominant, telomeric variant surface glycoprotein ( VSG ) gene [3] as part of a polycistronic transcription unit. Pol-I transcription initiates at several sites but this is attenuated at all but one site [6] . T. brucei can switch to activate a new telomeric VSG expression site (ESs) but, significantly, switching occurs at low-frequency and all but one of the ESs typically remain ‘silent’, despite possessing all cis -elements required for expression [7] . The active VSG -ES is associated with an extranucleolar pol-I transcription factory, known as the expression site body (ESB) [8] , [9] . This VSG -ES is depleted of nucleosomes [10] , [11] and nuclease-hypersensitive chromatin persists at this locus even if transcription is blocked [12] . An HMG chromatin protein is enriched at both the ESB and the nucleolus [12] , [13] , and a focus of SUMOylation associates with the ESB [14] . In addition, histones [15] and histone variants [16] , telomere-binding proteins, a histone H3-K76 methyltransferase, a histone deacetylase, a chromatin remodeler, histone chaperones, nuclear lamina components, cohesin and the inositol phosphate pathway all impact VSG -ES silencing to varying degrees (reviewed in ref. [17] ). These factors may impact chromatin-dependent silencing or transcriptional permissivity but, notably, a direct role in gene selection has not been demonstrated. More recently, the first factor specifically enriched in association with the active VSG -ES, VSG exclusion 1 (VEX1), was identified [17] . Here, we identify and characterise a VEX1–VEX2 complex. The complex assembles a sub-nuclear domain in a transcription-dependent manner and maintains VSG allelic exclusion by negatively controlling transcription of other telomeric VSGs . Inheritance of VSG exclusion requires maintenance of the VEX-complex during S-phase, which depends upon the conserved chromatin assembly factor, CAF-1. A subtelomere- and VSG -associated VEX-complex We previously described T. brucei VEX1 (Tb927.11.16920), the only known protein specifically enriched in association with the ESB [17] . VEX1, therefore, is at the heart of the nuclear subdomain meditating antigenic variation in trypanosomes, but VEX1 lacks orthologs in other cell types, it remained unclear why VSG -exclusion was only partially perturbed following VEX1-knockdown and it remained unclear whether other factors were involved in VSG -exclusion. To identify VEX1 chromatin interactions, we affinity-purified VEX1 myc -associated chromatin and deep-sequenced the enriched DNA. Reads were accurately aligned to individual VSG -ESs by uniqueness filtering, using MapQ > 1 [18] . An examination of protein coding sequences within the hemizygous subtelomeric VSG- ESs [7] , [19] revealed VSG-2 , the active VSG , as the most enriched gene (Fig. 1a , Supplementary Data 1 , sheet 1). We also observed particularly strong enrichment of the region downstream of this gene (Fig. 1a ). This is consistent with a focus of VEX1 that is adjacent to, rather than coincident with, the extranucleolar focus of pol-I at the active VSG -ES [17] . Notably, DNA immediately downstream of several silent ES-associated VSGs was also enriched (Fig. 1a , Supplementary Fig. 1 ). This is also consistent with our model proposing that conserved VSG -associated sequences, including the telomeric repeats, participate in VEX1- and homology-dependent VSG -silencing [17] . Thus, chromatin interactions connect VEX1 to the conserved sequences associated with telomeric VSGs . Fig. 1 A subtelomere- and VSG -associated VEX-complex. a Affinity purification of VEX1 myc -associated chromatin followed by sequencing (ChIP-seq). Enrichment traces over active ( VSG-2 ) and silent ( VSG-6 , VSG-13 ) VSG -ESs with 1 kbp non-overlapping bins; red circles, promoters; red boxes, VSGs ; grey boxes, expression-site associated genes ( ESAGs ). Box-plot depicting enrichment of the indicated CDSs. Centre lines show the medians; box limits indicate the 25th and 75th percentiles; whiskers extend from the 10th to the 90th percentile, outliers are shown. Silent VSGs , n = 18; ESAGs , n = 129. Metagene plot and the associated heat-map for active and silent telomeric VSGs . The red bar on the metagene plot indicates the location of a highly conserved sequence in the VSG 3’-untranslated region. b VEX1 GFP immunoprecipitation and proteomics. GFP-tag dependent enrichment from bloodstream form T. brucei . emPAI, exponentially modified protein abundance index. The inset shows immunoprecipitates and tag-dependent VEX1 (red) and VEX2 (green) bands highlighted in a silver-stained gel. c Schematic representation of VEX1 (Tb927.11.16920), VEX2 (Tb927.11.13380) and CAF-1 subunits (a, Tb927.8.3980; b, Tb927.10.7050; c, Tb927.11.4970) indicating conserved domains and motifs. d Immunofluorescence analysis during the cell cycle and protein-blot analysis of myc VEX2 expression. N nucleus; K kinetoplast (mitochondrial genome). e , f Immunofluorescence-based colocalisation studies of VEX2 GFP and VEX1 myc ( e ) or a nucleolar (No) and ESB marker (pol-I, largest subunit), a nucleolar marker (NOG1) or Histone H3 ( f ). In e , G1 or G2 cells are shown. d – f DNA was counter-stained with DAPI; the images correspond to maximal 3D projections of 0.1 μm stacks; scale bars 2 μm; the data are representative of independent biological replicates and independent experiments. Source data are provided as a Source Data file Full size image Next, we affinity-purified VEX1 GFP -associated proteins using cryomilling and high-affinity nanobodies. The procedure was carried out initially in insect-stage T. brucei (Supplementary Fig. 2a, b ), for which protocols were established [20] , and then in bloodstream form T. brucei (Fig. 1b ). Quantitative proteomic analysis (Fig. 1b , Supplementary Fig. 2a, b , Supplementary Data 1 , sheet 2) revealed tag-dependent enrichment of green flourescent protein (GFP) and the same set of five proteins in four independent experiments; VEX1 was enriched, as expected, but also Tb927.11.13380, an ortholog of the nonsense-mediated mRNA-decay ATP-dependent superfamily 1-type helicases, UPF1/SMG2/NAM7/Rent1 [21] , (Fig. 1c , Supplementary Fig. 2c–e ), now designated VEX2 (predicted 224 kDa, 2026 residues). Trypanosomes encode two UPF1-related proteins (Supplementary Fig. 2c ). The putative T. brucei canonical UPF1 has been studied but it remains unclear whether classical nonsense-mediated decay operates [22] . VEX2 contains a UPF1-related helicase domain towards the C -terminus, including the canonical motifs involved in ATP binding and hydrolysis and nucleic acid binding (Supplementary Fig. 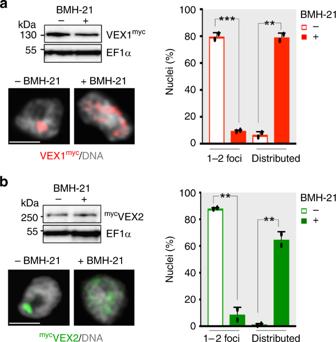Fig. 2 VEX-complex compartmentalisation is transcription dependent.a,bProtein-blot and immunofluorescence analysis of VEX1myc(a) andmycVEX2 (b) before and after BMH-21 treatment (30 min at 1 μM). Proportions of nuclei displaying 1–2 major foci or distributed signals are indicated; the remaining cells displayed no detectable signal. Values are averages of two independent experiments (≥100 nuclei each). Error bars, SD; **p< 0.01; ***p<0.001 (two-tailed paired Student’sttest). DNA was counter-stained with DAPI; the images correspond to maximal 3D projections of 0.1 μm stacks; scale bars 2 μm; the data are representative of independent biological replicates and independent experiments. Source data are provided as a Source Data file 2d ). Structural prediction suggested the presence of an α-solenoid architecture at the N -terminus (Supplementary Fig. 2e ), in place of the typical UPF2-interacting domain [23] ; α-solenoids are frequently involved in protein–protein or protein–RNA interactions. The other three proteins that displayed tag-dependent enrichment were all three components of chromatin assembly factor 1 (CAF-1; CAF-1a, Tb927.8.3980; CAF-1b, Tb927.10.7050, CAF-1c, Tb927.11.4970; Fig. 1b, c , Supplementary Fig. 2a ), the evolutionary conserved hetero-trimeric replication-associated histone chaperone [24] . Notably, no pol-I components were enriched. Super-resolution fluorescence microscopy revealed that, like VEX1, VEX2 localised to a single major sub-nuclear focus (detected in ~80% of nuclei) that was replicated and segregated at the appropriate phases of the cell cycle (Fig. 1d ). Consistent with the proteomics evidence, VEX2-foci co-localised with VEX1 foci (Fig. 1e , Supplementary Movie 1 ) and the extranucleolar, histone-depleted pol-I compartment (Fig. 1f ). We conclude that the VEX1–VEX2-complex is associated with the single VSG transcription compartment. VEX-complex compartmentalisation is transcription-dependent VEX1 foci are disrupted in cells treated with transcription inhibitors, indicating that active transcription is required for assembly [17] , [25] . However, it was unclear from these studies whether VEX1 was degraded or redistributed throughout the nucleoplasm. Protein blotting indicated that neither VEX1 (Fig. 2a ) nor VEX2 (Fig. 2b ) were degraded following pol-I specific transcription inhibition with BMH-21. Indeed, super-resolution confocal microscopy revealed that both VEX1 (Fig. 2a , Supplementary Fig. 3a ) and VEX2 (Fig. 2b , Supplementary Fig. 3b ) displayed significant levels of redistribution across the nucleus following inhibition of pol-I transcription, or inhibition of general transcription with actinomycin D (Supplementary Fig. 3c–f ). Thus, recruitment of VEX1 and VEX2 to the VSG transcription compartment requires active pol-I transcription. VEX1 and VEX2 proteins remain within the nucleus when transcription is prevented, suggesting availability for retargeting once pol-I transcription reinitiates. Fig. 2 VEX-complex compartmentalisation is transcription dependent. a , b Protein-blot and immunofluorescence analysis of VEX1 myc ( a ) and myc VEX2 ( b ) before and after BMH-21 treatment (30 min at 1 μM). Proportions of nuclei displaying 1–2 major foci or distributed signals are indicated; the remaining cells displayed no detectable signal. Values are averages of two independent experiments (≥100 nuclei each). Error bars, SD; ** p < 0.01; *** p < 0.001 (two-tailed paired Student’s t test). DNA was counter-stained with DAPI; the images correspond to maximal 3D projections of 0.1 μm stacks; scale bars 2 μm; the data are representative of independent biological replicates and independent experiments. Source data are provided as a Source Data file Full size image VEX2 depletion results in multi-VSG expression VEX1 was initially identified from a high-throughput RNA interference (RNAi) screen for subtelomeric loss-of-silencing [17] . Another genome-wide RNAi screen indicated minimal fitness-cost following VEX1-knockdown, but a significant and major fitness-cost following VEX2-knockdown, specifically in bloodstream-form cells and not insect-stage cells [26] (Supplementary Fig. 4a ). This likely explains why only VEX1, and not VEX2, was identified in the loss-of-silencing screen, and indicates a bloodstream-form specific function for VEX2; VSG is not normally expressed in the insect-stage. To explore the function of VEX2, we assembled three independent inducible RNAi knockdown strains with an active VSG-2 expression site (Fig. 3 , Supplementary Fig. 4b ). Knockdown was associated with a significant growth defect (Fig. 3a ), but little perturbation of cell cycle distribution (Supplementary Fig. 4c ). In these cells, normally silent VSG-6 was strongly derepressed after only 24 h, as assessed by protein immunoblotting (Fig. 3b ), immunofluorescence microscopy (Fig. 3c ) and immunostaining followed by flow cytometry (Fig. 3d ). Notably, abundance of the initially active VSG was also clearly reduced after 48 h of VEX2-knockdown (Fig. 3b ) and VSG-6 appeared to accumulate in intracellular compartments as well as at the surface (Fig. 3c , right-hand side). To survey additional VSGs, we used quantitative proteomics of proteins released from the cell-surface. The active VSG on wild-type cells, VSG-2, displayed a relative abundance of 99.9%. Following VEX2-knockdown, VSG-2 remained the most abundant VSG, but VSG-6 and several additional ES-associated VSGs were derepressed (Fig. 3e , Supplementary Data 1 , sheet 3). Because antigenic variation occurs at low frequency, T. brucei clones are typically homogeneous and express a single VSG (Fig. 3c–e ). Following VEX2-knockdown, however, >90% of cells simultaneously expressed VSG-2, and VSG-6 at the cell surface as determined by microscopy (Fig. 3c ) and flow cytometry (Fig. 3d ). Taken together, these results indicate major disruption of allelic exclusion and the simultaneous expression of multiple VSGs on the surface of individual cells following VEX2-knockdown. Fig. 3 VEX2 depletion results in multi-VSG expression. a Cumulative growth following tetracycline (Tet) induced VEX2-knockdown; * p < 0.05; ** p < 0.01 (multiple t tests). Protein blotting ( b ), immunofluorescence analysis ( c ), and flow cytometry ( d ), to assess VSG expression following VEX2-knockdown (24 h). EF1α, loading-control in ( b ); in c , DNA was counter-stained with DAPI and the graph depicts the rapid increase of dual VSG expressing cells following VEX2 knockdown by microscopy analysis. Scale bars, 5 μm (left hand side) and 2 μm (right hand side). Percentages in d indicate double-positive cells. e Quantitative mass spectrometry analysis of surface-VSGs following VEX2-knockdown (48 h). The inset shows data for wild-type cells. emPAI, exponentially modified Protein Abundance Index. Error bars (not visible in a ), SD; data are averages from two ( a / c / e ) independent biological replicates and representative of independent experiments ( a – d ). Source data are provided as a Source Data file Full size image VEX2 coordinates allele-specific VSG-ES transcription To further explore gene expression defects following VEX2-knockdown, we analysed the transcriptome, comparing three independent knockdown strains to three wild-type sub-clones (Supplementary Fig. 5 , Supplementary Data 1 , sheets 4–5). Since RNAi may not degrade the entire mRNA, we show efficient disruption of VEX2 transcript in Fig. 4a . Among approximately 7600 genes encoded in the genome, 166 displayed >5-fold and significantly ( p < 10 −2 ) increased expression after 24 h knockdown (Fig. 4b–e ), including every known pol-I transcribed protein-coding locus. There are 18 known silent, telomeric, pol-I promoter-associated VSGs in the genome; 13 in polycistronic expression sites and 5 in monocistronic expression sites, with the latter only normally activated in metacyclic cells in the insect salivary gland [18] . Total transcript abundance from this full set of 18 VSGs (Fig. 4b, c ), and 130 silent expression-site associated genes ( ESAGs ) (Fig. 4d ), was increased by 212 and 32-fold, respectively. Even the ESAGs at the active transcribed locus ( n = 18) were significantly ( p < 10 −50 ) upregulated (9-fold, Fig. 4d ), as were the non-telomeric, pol-I transcribed procyclin (associated) genes (Fig. 4e ); procyclin genes produce abundant surface proteins that are normally expressed only in insect mid-gut stage cells. Highlighting the magnitude of the VEX2-knockdown phenotype, derepressed VSGs contributed >24% of total VSG transcripts, compared to only 0.1% in control cells (Supplementary Data 1 , sheets 4–5); the super-abundant active VSG mRNA is >200-fold more abundant than the average mRNA encoding ribosomal proteins. Notably, several previously silent VSGs in ESs with dual promoters ( VSG-6, 8, 15 and 17 ; see ref. [7] ) were particularly derepressed and produced the four most abundant cellular mRNAs, after VSG-2 ; these VSGs were also readily detected at the cell-surface following VEX2-knockdown (Fig. 3e ). The same VSG -ESs were activated at high rates during VSG switching [27] . Thus, an additional VSG -ES promoter likely facilitates the derepression or activation of a VSG -ES. We conclude that VEX2 coordinates VSG allelic exclusion and has a profound impact on differential VSG expression. Fig. 4 VEX2 coordinates allele-specific VSG-ES transcription. a – e RNA-seq analysis following VEX2-knockdown (24 h). Total number of reads at VEX2 locus in the parental population or following VEX2 RNAi (target fragment indicated) ( a ). b – e Values are averages from three independent RNAi strains relative to wild-type controls and numbers in brackets indicate increase in transcript abundance for each gene cohort. Red square, VSG-2 ; black circle, VEX2 . Lower panels show transcript abundance at the silent VSG-6 , active VSG-2 and procyclin loci, respectively. Red circles, promoters; red boxes, VSGs ; grey boxes, other genes. RPKM/RPM, reads per (kilobase per) million. f Immunofluorescence and protein-blot analysis of pol-I expression and localisation following VEX2 RNAi. The bar graph indicates the proportion of nuclei ( n ≥ 100) with nucleolar and/or extranucleolar pol-I signals; the remaining cells displayed no detectable signal. DNA was counter-stained with DAPI; the images correspond to maximal 3D projections of 0.1 μm stacks; scale bars 2 μm. Error bar, SD; * p < 0.05; ** p < 0.01 (two-tailed paired Student’s t test); data are averages from three independent biological replicates and representative of independent experiments. Source data are provided as a Source Data file Full size image We did not anticipate increased expression of ESAGs at the active VSG -ES in response to VEX2-knockdown (Fig. 4d ). However, it has long been known that ESAGs upstream of VSGs , despite co-transcription in the same polycistron, yield far less abundant transcripts, and no factor responsible for this differential control had been identified previously; VSG mRNA is >140-fold more abundant than the mean ESAG mRNA [18] . Our transcriptome analysis now indicates post- or co-transcriptional suppression of these ESAGs mediated by VEX2. We speculate, based on sequence similarity of VEX2 to UPF1, that negative control by VEX2 may be related to nonsense-mediated mRNA-decay. We next asked what impact VEX2-knockdown and VSG -ES derepression had on RNA pol-I localisation. Immunofluorescence microscopy revealed a remarkable loss of the nucleolar pol-I signal after only 24 h of knockdown and a substantial loss of detectable extranucleolar pol-I foci; protein blotting indicated that pol-I was still present following VEX2 knockdown (Fig. 4f ). These results suggest that derepressed VSG -ESs deplete the nucleolus and the ESB of pol-I, redistributing the polymerase to multiple extranucleolar sites. VEX-complex knockdown yields a severe exclusion defect VEX1 knockdown yielded a moderate VSG derepression defect [17] relative to the VEX2 knockdown phenotype (Figs. 3 and 4 ). We, therefore, knocked down both VEX1 and VEX2 simultaneously and carried out a similar analysis to that described above. VEX1–VEX2 double knockdown was associated with a very severe growth defect that was cytocidal after 72 h (Fig. 5a ). In these cells, silent VSG-6 was again strongly derepressed, as assessed by protein immunoblotting; the active-VSG signal was once again clearly reduced after 48 h of knockdown (Fig. 5b ). Following 48 h of VEX1–VEX2 double knockdown, immunofluorescence microscopy revealed that almost all cells expressed both VSG-2 and VSG-6, while >20% of cells simultaneously expressed VSG-2, VSG-6 and VSG-3 (Fig. 5c ); VSG-13 was also expressed by >20% of these cells (Supplementary Fig. 6a ). We further monitored VEX1-knockdown cells over an extended period, during which cells remain viable [17] . This revealed >25% of the population expressing both VSG-2 and VSG-6 throughout the time-course, with no evidence for switching to VSG-6 expression (Supplementary Fig. 6b ). Thus, VEX-complex knockdown disrupts allelic exclusion and does not simply increase the VSG switching rate. Quantitative proteomic analysis following VEX1–VEX2 knockdown revealed derepression of 15 pol-I promoter-associated VSGs (Fig. 5d , Supplementary Data 1 , sheet 3). A comparison of relative VSG expression revealed that derepressed VSGs contributed approx. 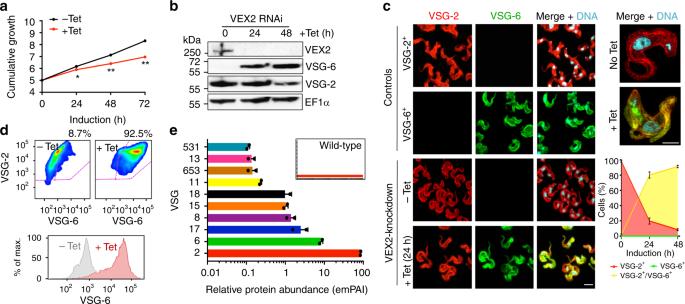Fig. 3 VEX2 depletion results in multi-VSG expression.aCumulative growth following tetracycline (Tet) induced VEX2-knockdown; *p< 0.05; **p< 0.01 (multiplettests). Protein blotting (b), immunofluorescence analysis (c), and flow cytometry (d), to assessVSGexpression following VEX2-knockdown (24 h). EF1α, loading-control in (b); inc, DNA was counter-stained with DAPI and the graph depicts the rapid increase of dual VSG expressing cells following VEX2 knockdown by microscopy analysis. Scale bars, 5 μm (left hand side) and 2 μm (right hand side). Percentages indindicate double-positive cells.eQuantitative mass spectrometry analysis of surface-VSGs following VEX2-knockdown (48 h). The inset shows data for wild-type cells. emPAI, exponentially modified Protein Abundance Index. Error bars (not visible ina), SD; data are averages from two (a/c/e) independent biological replicates and representative of independent experiments (a–d). Source data are provided as a Source Data file 40% of total VSG following VEX1–VEX2 knockdown (Fig. 5e , Supplementary Data 1 , sheet 3) compared to only approximately 10% of total VSG following VEX2 knockdown. As for VEX2-knockdown (Fig. 4f ), double knockdown was associated with loss of both the nucleolar pol-I signal and detectable extranucleolar pol-I foci (Supplementary Fig. 6c ). Fig. 5 VEX-complex knockdown yields a severe exclusion defect. a Cumulative growth following tetracycline (Tet) induced VEX1-VEX2 double knockdown; * p < 0.05; ** p < 0.01 (multiple t tests). Protein blotting ( b ), and immunofluorescence analysis ( c ), to assess VSG expression following VEX1–VEX2 double knockdown (24 h). Other details as in Fig. 3a–c . In c , an additional silent VSG, VSG-3, was analysed. d Quantitative mass spectrometry analysis of surface-VSGs following VEX1-VEX2 double knockdown (48 h). The inset shows data for wild-type cells. e Relative abundance of surface-VSGs following VEX2 or VEX1/VEX2-knockdown (48 h). emPAI, exponentially modified Protein Abundance Index ( d , e ). Data are averages from two independent biological replicates ( a , c – e ) and representative of independent experiments ( a – c ). Error bars, SD. f – j RNA-seq analysis following VEX1–VEX2 double knockdown (24 h). Total number of reads across VEX1 and VEX2 loci in the parental population or following knockdown ( f ). In g – j specific cohorts of genes are highlighted and values are averages from three independent RNAi strains relative to wild-type controls. Numbers in square brackets indicate increase in total transcript abundance for each category; RPKM, reads per kilobase per million. Source data are provided as a Source Data file Full size image Transcriptome analysis following VEX1–VEX2 knockdown (Fig. 5f , Supplementary Fig. 7 , Supplementary Data 1 , sheets 4–5) revealed a similar pattern of derepression as observed above for VEX2 knockdown alone (Fig. 5g–j ). Again, all known pol-I transcribed protein-coding loci were derepressed, and previously silent VSGs linked to dual VSG -ES promoters produced the four most abundant cellular mRNAs, after VSG-2 (Fig. 5g ). These data demonstrate that the VEX-complex coordinates VSG allelic exclusion. The allelic exclusion system collapses following depletion of the VEX-complex, yielding multi- VSG expression, highly heterogeneous VSG coats and cell-death. VEX-complex interactions impact abundance and location We next asked what impact VEX1 and VEX2 have on each other. VEX1-knockdown had no detectable impact on VEX2 expression or focal localisation (Fig. 6a ). In contrast, VEX1 over-expression substantially diminished VEX2 abundance; VEX1 was highly overexpressed in most nuclei (~80%) and VEX2 foci were no longer detectable by immunofluorescence (Fig. 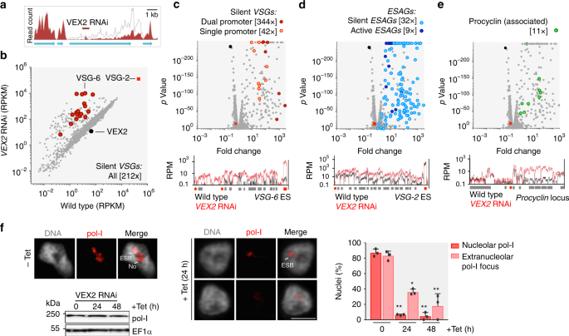Fig. 4 VEX2 coordinates allele-specificVSG-EStranscription.a–eRNA-seq analysis following VEX2-knockdown (24 h). Total number of reads atVEX2locus in the parental population or followingVEX2RNAi (target fragment indicated) (a).b–eValues are averages from three independent RNAi strains relative to wild-type controls and numbers in brackets indicate increase in transcript abundance for each gene cohort. Red square,VSG-2; black circle,VEX2. Lower panels show transcript abundance at the silentVSG-6, activeVSG-2and procyclin loci, respectively. Red circles, promoters; red boxes,VSGs; grey boxes, other genes. RPKM/RPM, reads per (kilobase per) million.fImmunofluorescence and protein-blot analysis of pol-I expression and localisation following VEX2 RNAi. The bar graph indicates the proportion of nuclei (n≥ 100) with nucleolar and/or extranucleolar pol-I signals; the remaining cells displayed no detectable signal. DNA was counter-stained with DAPI; the images correspond to maximal 3D projections of 0.1 μm stacks; scale bars 2 μm. Error bar, SD; *p< 0.05; **p<0.01 (two-tailed paired Student’sttest); data are averages from three independent biological replicates and representative of independent experiments. Source data are provided as a Source Data file 6b ). These data likely explain the previously reported more severe VSG derepression phenotype following VEX1 over-expression compared with knockdown [17] and also indicate that VEX1 can limit VEX2 abundance; this latter feature may be important for preventing activation of a second VSG . We also tested the impact of VEX2-knockdown on VEX1 localisation and found that VEX1 was redistributed across multiple sub-nuclear puncta following loss of VEX2 (Fig. 6c ). Thus, VEX1 association with the VSG transcription compartment is VEX2-dependent. Fig. 6 VEX-complex interactions impact abundance and location. a , b Protein-blot and immunofluorescence analysis following Tet-induced VEX1 knockdown and Tet-induced myc VEX1 overexpression, respectively (48 h). In the upper immunofluorescence panels, cells were stained with α-VSG-2 and α-VSG-6 to confirm the dual VSG expression phenotypes reported previously [17] . In the lower panels, cells were stained with α-myc for VEX2 localisation ( a ) or both α-myc and α-GFP for VEX1 and VEX2 localisation, respectively ( b ). The bar graphs indicate the proportion of ≥300 nuclei with 1–2 myc VEX2 foci following 48 h of VEX1 knockdown ( a ) or with 1–2 GFP VEX2 foci following 48 h of VEX1 overexpression ( b ). The proportion of nuclei displaying a distributed VEX1 signal (due to overexpression) is also shown in b ; the remaining cells displayed no detectable signal. c Protein-blot and immunofluorescence analysis of VEX1 Myc following Tet-induced VEX2 knockdown (24 h). The bar graph indicates the proportion of nuclei with 1–2 VEX1 myc foci or distributed signal, the remaining cells displayed no detectable signal. The bean-plot shows signal intensity in ≥100 nuclei with 1–2 major VEX1 myc foci (−Tet) or nuclei with a distributed signal (+Tet 24 h) following VEX2 knockdown. Black lines show the medians; pink/red lines represent individual data points; polygons represent the estimated density of the data. CTNF corrected total nuclear fluorescence, normalised to the nuclear area. EF1α was used as a loading-control. DNA was counter-stained with DAPI; scale bars 2 μm. The images in ( c ) correspond to maximal 3D projections of 0.1 μm stacks. For bar graphs, data representative of independent experiments and averages from two independent biological replicates; error bars, SD. ns, non-significant; * p < 0.05; *** p < 0.001; **** p < 0.0001 (two-tailed paired and unpaired Student’s t tests applied to bar graphs and bean plot, respectively). Source data are provided as a Source Data file Full size image VEX-complex compartmentalisation is stage-specific Insect-stage T. brucei cells neither transcribe VSG nor exhibit allelic exclusion. Since we show above that VEX-complex association with the VSG transcription compartment requires pol-I transcription, we asked whether VEX2 association with this compartment is absent in insect-stage cells. Like VEX1 [17] , VEX2 was indeed redistributed through the nuclear compartment during differentiation (Fig. 7a ). Protein blotting revealed substantial upregulation of VEX2 as the VSG signal diminished (Fig. 7a ) and these differentiated cells displayed multiple VEX2-foci, some of which were coincident with VEX1-foci (Fig. 7b ). Redistributed VEX2 was similarly observed in long-term established insect-stage cells. Thus, both VEX1 and VEX2 associate with the VSG transcription compartment in a pol-I transcription-dependent and life cycle stage-specific manner. Fig. 7 VEX-complex compartmentalisation is stage-specific. a Immunofluorescence and protein-blot analysis of myc VEX2 localisation and expression, respectively, following differentiation of bloodstream forms (BSFs, 0 h) into procyclic forms (PCFs). As immunofluorescence control, the cells were stained for the major surface glycoprotein for each developmental stage; VSG in BSFs and EP-procyclin in PCFs. For protein blotting, EF1α was used as a loading-control. b GFP VEX2/VEX1 myc colocalisation studies in 48 h differentiated BSFs. In b , these images correspond to maximal 3D projections of 0.1 μm stacks. DNA was counter-stained with DAPI; scale bars 2 μm. Data representative of independent experiments. Source data are provided as a Source Data file Full size image Colocalisation of CAF-1 and the VEX-complex during S phase We next considered the interaction between the VEX-complex and CAF-1; all three components of this conserved chromatin chaperone were co-immunoprecipitated with VEX1 (see Fig. 1b ). DNA replication presents both an opportunity to retain or reset epigenetic states. We, therefore, asked if CAF-1 plays a role in the inheritance of the VEX-complex-dependent epigenetic state during DNA replication; the active VSG -ES is replicated early during S-phase while the silent VSG -ESs are replicated later [28] . Significantly, S-phase specific VSG- ES derepression was previously reported following CAF-1b knockdown [15] . By analysing the localisation of a tagged CAF-1b subunit, either CAF-1b GFP or CAF-1b myc , we observed major CAF-1b foci, despite an overall punctate nuclear distribution. Notably, these foci co-localised with the sub-nuclear compartment defined by both VEX1 (Fig. 8a , Supplementary Movie 2 ) and VEX2 (Fig. 8b ) and coincident signals were significantly enriched in S-phase cells (Fig. 8a, b ); the interaction between the VEX-complex and CAF-1 was also confirmed by immunoprecipitation followed by protein blotting (Fig. 8c ). Fig. 8 Colocalisation of CAF-1 and the VEX-complex during S phase. a , b Immunofluorescence-based colocalisation studies of VEX1 myc /CAF-1b GFP and VEX2 GFP /CAF-1b myc . Representative images from G1 and S phase cells are shown. Nuclei ( n ≥ 70) were scored for CAF-1b puncta coincident with VEX1 myc /VEX2 GFP foci. DNA was counter-stained with DAPI; scale bars, 2 μm. Error bars, SD; * p < 0.05; ** p < 0.01; *** p < 0.001 (one-way ANOVA test). Values are averages from two independent biological replicates and are representative of independent experiments. The images on the right-hand side correspond to maximal 3D projections of 0.1 μm stacks. c Co-immunoprecipitation of VEX2 GFP /CAF-1b myc followed by protein-blot analysis. Green circle, GFP; black circles, myc; I, input; E, elution. Source data are provided as a Source Data file Full size image VEX-complex reassembly and inheritance requires CAF-1 By analysing phenotypes associated with CAF-1b knockdown, we confirmed two further specific predictions in support of CAF-1 dependent inheritance of the VEX-complex. First, VEX1 distributed across multiple sub-nuclear puncta following CAF-1b knockdown (12 h, Fig. 9a ); while VEX2 notably remained primarily compartmentalised in a single focus in each nucleus under the same conditions (Fig. 9b ). Indeed, we observed more intense VEX2 foci following CAF-1b knockdown, and protein blotting confirmed that VEX2 abundance is specifically increased when CAF-1b is depleted (Fig. 9c , Supplementary Fig. 8a, b ). Thus, CAF-1 limits VEX2 abundance, an effect that may be enhanced by excess VEX1 (see above). Second, following CAF-1b knockdown (see Fig. 9d ), transcriptome analysis revealed specific derepression of VSGs and other pol-I transcribed protein-coding genes (Fig. 9e–i , Supplementary Fig. 8c, d , Supplementary Data 1 , sheets 4–5). Fig. 9 VEX-complex reassembly and inheritance requires CAF-1. VEX1 myc ( a ), but not myc VEX2 ( b ), is distributed following tetracycline (Tet) induced CAF-1b knockdown (12 h), as assessed by immunofluorescence analysis. DNA was counter-stained with DAPI; scale bars, 2 μm. The images correspond to maximal 3D projections of 0.1 μm stacks. Error bars, SD; ns, not significant; ** p < 0.01 (two-tailed paired Student’s t test). Values are averages from three independent biological replicates and are representative of independent experiments (the remaining cells displayed no detectable signal). c Protein-blot analysis of CAF-1b myc , myc VEX2 and VEX1 myc expression following CAF-1b knockdown. EF1α was used as a loading-control. d – i RNA-seq analysis following CAF-1b knockdown (24 h). d Total number of reads across CAF-1b locus in the parental population or following CAF-1b RNAi. e – i Values are averages from two independent RNAi strains relative to wild-type controls. Panel e shows transcript abundance at the silent VSG-6 ES. Red circles, promoters; red boxes, VSGs ; grey boxes, other genes. RPKM/RPM, reads per (kilobase per) million ( e – i ). Panels f – i highlight different gene cohorts and numbers in square brackets indicate increase/decrease in total transcript abundance for each category; red square, VSG-2 ; black circle, CAF-1b . Promoter-proximal VSGs and ESAGs (6, 7 and 10) are within 5 kbp of a promoter, distal VSGs are 46 +/−4 kbp from the promoter. Source data are provided as a Source Data file Full size image Following CAF-1b knockdown for 24 h (see Supplementary Fig. 8c ), 115 genes displayed >5-fold and significantly ( p < 10 −2 ) increased expression, >80% of which were also significantly increased following VEX2 knockdown (Supplementary Data 1 , sheets 4, 5). In this case, we observed a more pronounced increase in total transcript abundance for promoter-proximal VSGs (89-fold, n = 5, Fig. 9g ) relative to promoter-distal VSGs (9-fold, n = 5, Fig. 9g ). Similarly, we observed a more pronounced increase in total transcript abundance for promoter-proximal ESAGs (48-fold, n = 34, Fig. 9h ) relative to promoter-distal ESAGs (4-fold, n = 96, Fig. 9h ). Procyclin (associated) genes were also derepressed (6-fold, Fig. 9i ), while ESAGs at the active locus displayed significantly ( p < 10 −4 ) reduced expression (44 ± 19%, n = 12; Fig. 9h , Supplementary Data 1 , sheets 4–5), consistent with increased VEX2 abundance and enhanced VEX2-mediated negative control at this locus (see above). Thus, CAF-1 knockdown has a major impact on pol-I transcribed protein-coding loci; promoter-proximal genes may be particularly susceptible to derepression due to a genome-wide histone chaperone defect. A model for VSG allelic exclusion by the VEX-complex Finally, combining RNA-seq data, we compared the relative contributions of VEX1, VEX2 and CAF1-b to VSG silencing (Fig. 10a ) and also calculated relative contributions to an allelic exclusion index; the ratio of reads from the active VSG relative to all 18 silent expression-site associated VSGs (Fig. 10b ). VEX2 clearly makes the major contribution to VSG silencing (Fig. 10a, b ), establishing a 1000-fold expression differential in wild-type cells, which, following VEX2 or VEX-complex depletion, is diminished to a 2–4-fold differential (Fig. 10b ). As illustrated by our model (Fig. 10c ), we conclude that the VEX-complex associates with the active VSG in a pol-I transcription-dependent manner and thereby coordinates nuclear pol-I compartments and VSG exclusion. VEX1 compartmentalisation is VEX2-dependent, while retention during DNA replication is also CAF-1 dependent. Fig. 10 A model for VSG allelic exclusion by the VEX-complex. a , b Comparative analysis of VSG -transcripts from wild-type T. brucei or following VEX1 (data from Glover et al., 2016; dashed boxes), VEX2, VEX1/VEX2 and CAF-1b knockdown (data from current study). a The box-plot depicts the sum of silent VSG expression; whiskers extend from the minimal to the maximal value, other details as in Fig. 1a . b The allelic exclusion index represents active VSG-2 expression divided by the expression of all other expression site associated VSGs combined. Error bars, SD. c A model for heritable exclusion by the VEX-complex and CAF-1. Left-hand panel: VSG -ES transcription drives competition for a limited pool of the VEX-complex. Once associated with chromatin, the complex promotes transcription and transmits a silencing signal, excluding other VSG -ESs, ultimately allowing only one VSG -ES to recruit sufficient pol-I and to form a pol-I transcription compartment. CAF-1 dependent compartmentalisation of the complex provides allele-specific epigenetic inheritance. Middle and right-hand panels: VEX2 or CAF-1 depletion disrupts the VEX-complex associated transcription compartment and the silencing signal; it remains unclear how VEX1 interacts with VSG -ESs under these circumstances. Bent arrows and dashed arrows indicate VSG -ES promoters and transcription, respectively. Source data are provided as a Source Data file Full size image An improved understanding of immune evasion by pathogens has profound importance to health and disease. Despite intense study, mechanisms underlying stochastic activation of one allele and the heritable exclusion of all others remain to be fully defined. This has been the case for antigenic variation in the parasites that cause malaria [1] , giardiasis [2] and African trypanosomiasis; [3] and also in mammals where olfactory receptor allelic exclusion underpins odour detection [4] and where immunoglobulin and receptor allelic exclusion underpin specificity in B and T cells [5] . Here, we describe an association between a bipartite VSG exclusion (VEX)-complex and the active VSG transcription sub-compartment in T. brucei . The complex, which is compartmentalised due to active VSG -ES transcription, mediates transcriptional silencing of all other VSG alleles (Fig. 10c ). In addition, VEX1 sequestration requires VEX2, and also CAF-1 during DNA replication. Transcription-dependent sequestration, and a major allelic exclusion defect when the VEX-complex is depleted are consistent with a sequestration-transcription based positive-feedback mechanism, favoring sequestration of the VEX-complex at the transcribed VSG compartment. This may be important for maintaining, and we speculate, also establishing, allelic exclusion. CAF-1 dependence indicates that inheritance of exclusion requires VEX1 reloading during, or soon after, DNA replication. Notably, the VEX-complex is also present in insect-stage cells, suggesting availability for retargeting once VSG transcription reinitiates in parasites in the insect salivary gland. Several observations suggest potentially shared mechanisms with allelic exclusion in mammals. The VEX2-related UPF1 orthologue in humans (Rent1) influences early nuclear events in mRNA biogenesis, including splicing [29] . Mammalian Rent1 is enriched at telomeres and negatively controls the association between telomeric repeat-containing RNA (TERRA) transcripts and chromatin at these sites; it has been proposed that these transcripts promote heterochromatin assembly, similar to Xist RNA promotion of X-chromosome inactivation [30] . In addition, murine UPF1 is required for X-inactivation and formation of Xist RNA domains, a function involving Xist splicing control [31] . Taken together, these findings suggest a conserved role for this helicase family in regulating lncRNA-chromatin associations, and possibly in gene expression choices. The enrichment of VEX1 and VEX2 in association with the active VSG -ES is also reminiscent of nuclear sub-structures in other eukaryotic cells, such as PML bodies and nuclear speckles [32] , [33] . It remains unclear how the activity state of a gene is reproduced on daughter chromatids following DNA replication. The conserved hetero-trimeric histone H3–H4 specific chaperone, CAF-1, participates in chromatin assembly directly behind the passing DNA polymerase during DNA replication, integrating DNA synthesis with conservative reassembly of chromatin in eukaryotes [24] , [34] . This involves reincorporating the majority of maternal histones within 400 bp of their pre-replication locus [35] and locus-specific bookmarking by epigenetic regulatory complexes to maintain transcriptional programs [36] , [37] . Mammalian CAF-1 sustains somatic cell types [38] and epigenetic memory by interacting with heterochromatin protein 1α, a histone H3 methyltransferase and KRAB-ZFP-associated protein 1; this complex is also associated with sub-nuclear foci [39] . Human CAF-1 can also activate transcription independent of its histone deposition function [40] and the conserved CAF-1 subunit-associated dREAM complex plays a role in specifying and maintaining olfactory receptor gene expression in Drosophila [41] . Thus, in addition to housekeeping roles in chromatin assembly, several lines of evidence suggest an evolutionary conserved role for CAF-1 in sustaining site-specific molecular memories of epigenetic states. Our findings indicate that this can involve CAF-1 dependent and locus-specific compartmentalisation of non-histone, chromatin-associated regulators as epigenetic marks. Consistent with this view, a cohesin-dependent delay in active VSG sister chromatid separation facilitates epigenetic inheritance [42] . Thus, premature segregation of sister chromatids following cohesin depletion may yield free VEX1 and present opportunities for activation of other VSG -ESs. VEX2 makes the greatest contribution to differential VSG expression, as assessed at mRNA and protein levels, while loss of both VEX1 and VEX2 leads to collapse of the exclusion system. Transcription sustains VEX-complex assembly at the active locus and this sequestration through transcription may also drive the establishment of a single active site. The VEX-complex may also be self-limiting, in the sense that CAF-1 and VEX1 can negatively control VEX2 expression; this may be important to minimise activation at other sites and hence secure selectivity. We previously demonstrated homology-dependent silencing by VEX1 [17] and suspect that communication among VSG alleles requires a trans -acting RNA component. Although the current findings demonstrate robust negative control of silent VSGs by the VEX-complex, a more detailed dissection of the proposed positive and negative controls, and their coordination to achieve allelic exclusion, will require further study. In summary, the crosstalk among VSG -ESs and inheritance of allelic exclusion in trypanosomes requires transcription, the VEX-complex and CAF-1 dependent partitioning of VEX1. These factors collectively sustain a specific assembly in association with the active VSG , resulting in exclusion of all other VSG alleles. CAF-1 links the VEX-complex to the active site to produce a molecular memory. Our findings reveal the factors underpinning a winner-takes-all paradigm for the establishment, maintenance and inheritance of nuclear bodies and allele-specific epigenetic states. To our knowledge, this is the first characterisation of a protein complex directly responsible for single gene choice in an allelic exclusion system. T. brucei growth and manipulation Bloodstream-form T. brucei , Lister 427 and 2T1 cells [43] , both wild-type with respect to VEX1, VEX2 and CAF-1 subunits, were grown in HMI-11 medium and genetically manipulated using electroporation [44] ; cytomix was used for all transfections. Puromycin, phleomycin, hygromycin and blasticidin were used at 2, 2, 2.5 and 10 µg ml −1 for selection of recombinant clones; and at 1, 1, 1 and 2 µg ml −1 for maintaining those clones, respectively. Cumulative growth curves were generated from cultures seeded at 10 5 cells ml −1 , counted on a haemocytometer and diluted back to 10 5 cells ml −1 as necessary. For differentiation of bloodstream form to procyclic form, 2 × 10 7 cells were resuspended in DTM medium, 2.5 mg ml −1 of haemin, 300 mM cis-aconitate and incubated at 27 °C. Established procyclic-form T. brucei , Lister 427 cells were grown in SDM-79 at 27 °C and genetically manipulated using electroporation as above. Blasticidin was used at 10 and 2 μg ml −1 for selection and maintenance, respectively. Plasmids For RNAi, primers were selected from ORF sequences using CLC Viewer v. 7.8 and BLAST analysis to minimise potential off-target effects. A specific RNAi target fragment for VEX2 (Tb927.11.13380, 471 bp) was amplified and cloned into pRPa iSL [45] . The VEX1 (Tb927.11.16920, 574 bp) [17] and CAF-1b (Tb927.10.7050, 458 bp) [15] RNAi cassettes were excised prior to electroporation by digesting with Asc I. For epitope-tagging at the native locus, a 710 bp fragment of VEX2 was amplified and cloned into pNAT TAGx [45] to add an N -terminal 6× c-myc or GFP-tag and a fragment of 918 bp was amplified and cloned into pNAT xTAG [45] to add a C -terminal GFP tag. The vectors were linearised with Xho I and Hpa I, respectively. The VEX1 12myc [17] and CAF-1b 12myc [15] C -terminal tagging vectors were linearised with Sph I and Nde I, respectively. The VEX1 and CAF-1b GFP C -terminal tagging vectors were made by replacing the 12× c-myc tag and were also linearised with Sph I and Nde I, respectively. The VEX1 C -terminal myc-tag overexpression cassette [17] was excised prior to electroporation by digesting with Asc I. Linearised RNAi and overexpression constructs, under the control of tetracycline-inducible promoters, were transfected into 2T1 cells, which allow for targeting to a single genomic locus validated for robust inducible expression [43] . ChIP-seq ChIP and cell lysis [46] was carried out with the following modifications. Briefly, 2 × 10 8 T. brucei bloodstream form cells expressing a C -terminal 12-myc tagged endogenous copy of VEX1 were cross-linked with 1% formaldehyde for 20 min at RT. DNA was sonicated using a Bioruptor (Diagenode) with sonication beads (Diagenode, C01020031) for 5 cycles of 30 s on/30 s off. C -terminal 12-myc VEX1 was immunoprecipitated with α-Myc antibody coupled to Dynabeads Protein G (2.8 µm). Antibody coupling to the Dynabeads was carried out according to the manufactures recommendations. The beads were then washed with RIPA buffer (50 mM HEPES-KOH, pKa 7.55, 500 mM LiCl, 1 mM EDTA, 1.0% NP-40, 0.7% Na-Deoxycholate) and eluted DNA was purified by phenol chloroform extraction and ethanol precipitation. Reads were mapped to bloodstream VSG -ESs [7] and metacyclic VSG- ESs [47] , [48] from the Lister 427 strain. Bowtie 2-mapping [49] was with the parameters --very-sensitive --no-discordant --phred33, and with a MapQ value of >1 [18] . Alignment files were manipulated with SAMtools [50] . 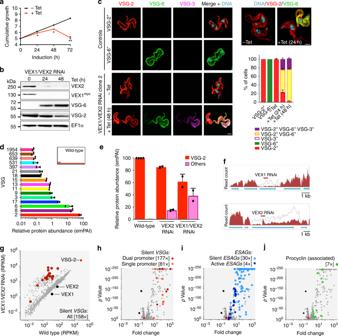Fig. 5 VEX-complex knockdown yields a severe exclusion defect.aCumulative growth following tetracycline (Tet) induced VEX1-VEX2 double knockdown; *p< 0.05; **p< 0.01 (multiplettests). Protein blotting (b), and immunofluorescence analysis (c), to assessVSGexpression following VEX1–VEX2 double knockdown (24 h). Other details as in Fig.3a–c. Inc, an additional silent VSG, VSG-3, was analysed.dQuantitative mass spectrometry analysis of surface-VSGs following VEX1-VEX2 double knockdown (48 h). The inset shows data for wild-type cells.eRelative abundance of surface-VSGs following VEX2 or VEX1/VEX2-knockdown (48 h). emPAI, exponentially modified Protein Abundance Index (d,e). Data are averages from two independent biological replicates (a,c–e) and representative of independent experiments (a–c). Error bars, SD.f–jRNA-seq analysis following VEX1–VEX2 double knockdown (24 h). Total number of reads acrossVEX1andVEX2loci in the parental population or following knockdown (f). Ing–jspecific cohorts of genes are highlighted and values are averages from three independent RNAi strains relative to wild-type controls. Numbers in square brackets indicate increase in total transcript abundance for each category; RPKM, reads per kilobase per million. Source data are provided as a Source Data file Alignments were inspected with the Artemis genome browser [51] . Telomeric VSG coding sequences with a mapping quality filtering of >1 were aligned using deeptools computeMatrix scale-regions. The bedgraph for log 2 fold change was generated using deepTools2 [52] with 1 kb bins and the option smoothLength 5000, plotted in Excel and further assembled in Illustrator. The heat map was generated using deepTools. Reads were counted using BEDTools [53] , counting reads in non-overlapping 1 kb bins. Files were normalised by counting total read counts per library prior to fold change calculation for each bin. Locus maps were generated by exporting vector graphics views or regions of interest from Artemis genome browser and manipulation in Adobe illustrator. The box plot was generated in Graphpad Prism v7.0. Affinity-enrichment of VEX1-interactors 1 × 10 10 insect or bloodstream form T. brucei cells with or without a C -terminal GFP-tagged endogenous copy of VEX1 were washed three times in ice cold PBS with protease inhibitors (Roche, EDTA free) and subsequently cryomilled into a fine grindate, in a planetary ball mill (Retsch) [20] ; protein–protein interactions are effectively preserved under these conditions. Six aliquots of 50 mg of frozen grindate were thawed into ice cold lysis buffer (20 mM HEPES, pH 7.4, 1 mM MgCl 2 , 10 µM CaCl 2 , protease inhibitor cocktail) containing either 100 mM NaCl or 250 mM citrate and either 0.1% Tween, 0.1% Brij58, 0.1% Triton X-100 or 0.1% Chaps, and pipetted to homogenise. The samples were then subjected to sonication (three pulses at 60% amp) and placed on ice. Samples were spun for 10 min at 20,000 g at 4 °C to pellet the debris. The supernatant was removed and added to a 1.5 ml eppendorf containing dimeric α-GFP nanobodies [54] conjugated to magnetic beads (Dynabeads—Thermo Scientific) and agitated at 4 °C for 2 h. The samples were then placed on a magnetic rack and washed three times with ice-cold lysis buffer. Samples were eluted with a non-reducing sodium dodecyl sulphate polyacrylamide gel electrophoresis (SDS-PAGE) loading buffer or equivalent. The resulting proteins were fractionated by 1D SDS-PAGE and visualised by silver staining. Quantitative mass spectrometry Affinity-enriched samples were run 2 cm into a NuPAGE ® Novex Bis–Tris 10% gel with NuPAGE ® MOPS SDS running buffer (Life Technologies) and subjected to overnight (16 h) trypsin digestion (Modified Sequencing Grade, Roche). Peptides were then extracted, dried in a SpeedVac (Thermo Scientific), resuspended in 50 µl 1% formic acid, centrifuged and transferred to high-performance liquid chromatography (HPLC) vials. 5 µl was typically analysed on a Q Exactive HF Hybrid Quadrupole-Orbitrap Mass Spectrometer (Thermo Scientific) coupled to an UltiMate 3000 RSLCnano ultra HPLC system (Thermo Scientific) and EasySpray column (75 μm × 50 cm, PepMap RSLC C18 column, 2 μm, 100 Å, Thermo Scientific). The mass spectrometer was operated in data dependent mode with a single MS survey scan from 335 to 1800 m / z followed by 20 sequential m/z dependent MS2 scans. The 20 most intense precursor ions were sequentially fragmented by higher energy collision dissociation. The MS1 isolation window was set to 1.4 Da and the resolution set at 60,000. MS2 resolution was set at 15,000. The AGC targets for MS1 and MS2 were set at 3e 6 ions and 2e 5 ions, respectively. The normalised collision energy was set at 27%. The maximum ion injection times for MS1 and MS2 were set at 50 and 19 ms, respectively. The peptides from each fraction were separated using a mix of buffer A (0.1% formic acid in MS grade water) and B (0.08% formic acid in 80% MS grade CH 3 CN) and eluted from the column using a flow rate of 300 nl min −1 and a linear gradient from 5 to 40% buffer B over 68 min. The column temperature was set at 50 °C. RAW data files were extracted and converted to Mascot generic files (.mgf) using MSC Convert. Data were searched against the MaxQuantTbrucei database using the Mascot Search Engine (Mascot Daemon Version 2.3.2). Fold-change, relative to a sample lacking GFP-tagged VEX1, was used to derive an enrichment score. For VSG analysis, glycosylphosphatidylinositol (GPI)-specific phospholipase C (GPI-PLC) cleaved soluble VSG (sVSG) was prepared and subjected to quantitative mass spectrometry analysis [17] , [55] ; the eluate was concentrated on an Amicon Ultra 0.5 ml centrifugal filter (Millipore), and recovered in 100 μl of water. emPAI scores are proportional to protein content in a protein mixture [56] . Co-Immuniprecipitation 4 × 10 8 bloodstream form T. brucei cells with or without a C -terminal GFP-tagged endogenous copy of VEX2 and a C -terminal 12-myc-tagged endogenous copy of CAF-1b were washed three times in ice-cold PBS with protease inhibitors and lysed into ice cold lysis buffer (RIPA, 1 mM DTT, protease inhibitor cocktail). Pipetting to homogenise, 30 s of vortexing and incubation for 30 min at 4 °C facilitated lysis. Samples were spun for 10 min at 20,000 g at 4 °C to pellet debris. The supernatant was removed and added to a 1.5 ml eppendorf containing α-GFP antibody (Abcam) conjugated to magnetic Dynabeads and agitated at 4 °C for 2 h. The samples were then placed on a magnetic rack and washed five times with ice-cold lysis buffer. Samples were eluted with a reducing NuPAGE LDS loading buffer. The resulting proteins were fractionated by 1D SDS-PAGE and analysed by protein-blotting. Protein blotting Protein samples were run according to standard protein separation procedures, using SDS-PAGE. However, for VEX2 detection, the use of Bis-Tris gels with a neutral pH environment and a bis–tris/bicine based transfer buffer (containing a reducing agent and 10% methanol) were critical for protein separation and transfer, respectively (NuPAGE, Invitrogen). Otherwise, western blotting was carried out according to standard protocols. The following primary antibodies were used: rabbit α-VEX2 (1:1000), rabbit α-pol-I largest subunit [17] (1:500), rabbit α-VSG-2 (1:20,000), rabbit α-VSG-6 (1:20,000), mouse α-c-myc (Millipore, clone 4A6, 1:7,000), rabbit α-GFP (Abcam, 1:1,000) and mouse α-EF1α (Millipore, clone CBP-KK1, 1:20,000). We used horseradish peroxidase coupled secondary antibodies (α-mouse and α-rabbit, Biorad, 1:2000). Blots were developed using an enhanced chemiluminescence kit (Amersham) according to the manufacturer’s instructions. Densitometry was performed using Fiji v. 2.0.0. Microscopy Immunofluorescence microscopy was carried out according to standard protocols, using 12-well 5 mm (Thermo Scientific) or 18-well μ-slides (Ibidi) for wide field, and confocal microscopy, respectively. For super-lowest speed; pinhol microscopy, the cells were attached to poly- l -lysine treated coverslips (#1.5), stained and only then mounted onto glass slides. For colocalisation studies with pol-I we used antigen-retrieval. Prior to permeabilization, fixed cells were rehydrated in phosphate-buffered saline (PBS) for 5 min at RT, held at 95 °C for 60 s in freshly prepared antigen-retrieval buffer (100 mM Tris, 5% urea, pH 9.5) and then washed 3 × 5 min in PBS at RT. Cells were mounted in Vectashield with DAPI (wide field) or stained with 1 µg ml −1 DAPI for 10 min and then mounted in Vectashield without DAPI (confocal and super resolution). In T. brucei , DAPI-stained nuclear and mitochondrial DNA were used as cytological markers for cell-cycle stage; one nucleus and one kinetoplast (1N:1K) indicates G1, one nucleus and an elongated kinetoplast (1N:eK) indicates S-phase, one nucleus and two kinetoplasts (1N:2K) indicates G2/M and two nuclei and two kinetoplasts (2N:2K) indicates post-mitosis [57] , [58] . Primary antisera were rat α-VSG-2 (1:10,000), rabbit α-VSG-6 (1:10,000), rabbit α-VSG-13 [59] (1:5000), mouse α-VSG-3 [60] coupled with Alexa 488 (1:500), mouse α-EP procyclin (Cedarlene, 1:1,000), rabbit α-GFP (Invitrogen, 1:250; Abcam, 1:500), mouse α-myc (Source Bioscience, clone 9E10, 1:200 or New England Biolabs, clone 9B11, 1:2,000), rabbit α-pol-I largest subunit [17] (1:100), rabbit α-NOG1 [61] (1:500) or rabbit α-histone H3 (Abcam, 1:1000). The secondary antibodies were Alexa Fluor conjugated goat antibodies (Thermo Scientific): α-mouse, α-rat and α-rabbit, AlexaFluor 488 or Alexa Fluor 568 (1:1000 or 1:2000, for confocal or wide field field microscopy, respectively) or α-rat Alexa 647 (1:1000). For the colocalisation studies in Fig. 8a, b and the quantification in Fig. 5c , cells were analysed by confocal microscopy, using a Leica TCS SP8 confocal laser scanning microscope and the Leica Application Suite X (LASX) software (Leica, Germany). For the remaining quantifications, cells were analysed by wide field microscopy, using a Zeiss Axiovert 200 M microscope with an AxioCam MRm camera and the ZEN Pro software (Carl Zeiss, Germany). The images were acquired as z -stacks (0.1–0.2 µm) and in the case of the wife field microscopy, further deconvolved using the fast iterative algorithm in Zen Pro. For all quantifications, images were acquired with the same settings and equally processed. Corrected total nuclear fluorescence = integrated density − (area of selected nucleus × mean fluorescence of background readings). Representative images were further acquired using a Leica TCS SP8 confocal laser scanning microscope in Hyvolution Mode and the Leica Application Suite X (LASX) software (Leica, Germany). The Hyvolution mode allows super-resolution level images, with settings: highest resolution/lowest speed; pinhole 0.5—Images with DNA in grey (or cyan); Figs. 1 d–f, 2 a, b, 3c (right hand side) 4 f, 5 c (right hand side), 6 c, 7 b, 8 a, b (right hand side), 9 a, b and Supplementary Fig. 3c, d . All the confocal images (with or without Hyvolution mode) correspond to maximal 3D projections by brightest intensity stacks of approximately 30 slices of 0.1 µm. All the images were processed, scored and the signal quantified using Fiji v. 2.0.0 [62] . Actinomycin D was applied at 10 µg ml −1 for 30 min and pol-I inhibitor (BMH-21) at 1 µM for 30 min, both at 37 °C. 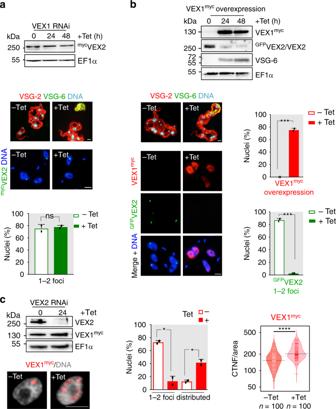Fig. 6 VEX-complex interactions impact abundance and location.a,bProtein-blot and immunofluorescence analysis following Tet-induced VEX1 knockdown and Tet-inducedmycVEX1 overexpression, respectively (48 h). In the upper immunofluorescence panels, cells were stained with α-VSG-2 and α-VSG-6 to confirm the dual VSG expression phenotypes reported previously17. In the lower panels, cells were stained with α-myc for VEX2 localisation (a) or both α-myc and α-GFP for VEX1 and VEX2 localisation, respectively (b). The bar graphs indicate the proportion of ≥300 nuclei with 1–2mycVEX2 foci following 48 h of VEX1 knockdown (a) or with 1–2GFPVEX2 foci following 48 h of VEX1 overexpression (b). The proportion of nuclei displaying a distributed VEX1 signal (due to overexpression) is also shown inb; the remaining cells displayed no detectable signal.cProtein-blot and immunofluorescence analysis of VEX1Mycfollowing Tet-induced VEX2 knockdown (24 h). The bar graph indicates the proportion of nuclei with 1–2 VEX1mycfoci or distributed signal, the remaining cells displayed no detectable signal. The bean-plot shows signal intensity in ≥100 nuclei with 1–2 major VEX1mycfoci (−Tet) or nuclei with a distributed signal (+Tet 24 h) following VEX2 knockdown. Black lines show the medians; pink/red lines represent individual data points; polygons represent the estimated density of the data. CTNF corrected total nuclear fluorescence, normalised to the nuclear area. EF1α was used as a loading-control. DNA was counter-stained with DAPI; scale bars 2 μm. The images in (c) correspond to maximal 3D projections of 0.1 μm stacks. For bar graphs, data representative of independent experiments and averages from two independent biological replicates; error bars, SD. ns, non-significant; *p< 0.05; ***p< 0.001; ****p< 0.0001 (two-tailed paired and unpaired Student’sttests applied to bar graphs and bean plot, respectively). Source data are provided as a Source Data file Flow cytometry Flow cytometry was carried out according to standard procedures. The primary antibodies were as follows: rat α-VSG-2 (1:10,000) and rabbit α-VSG-6 (1:10,000). Secondary antibodies were goat α-rat Alexa Fluor 647 and goat α-rabbit Alexa Fluor 488 (both 1:2000). DNA was stained with propidium iodide at 10 µg ml −1 . Samples were analysed on a BD LSRFortessa (BD Biosciences) and data were visualised using FlowJo software. More than 40,000 events were analysed to determine the percentage of cells in each quadrant. Transcriptome analysis RNA-seq analysis was performed using 2T1 cells and uninduced or induced clones of VEX2 (24 and 48 h), VEX1/VEX2 (24 and 48 h) or CAF-1b (24 h) RNAi. 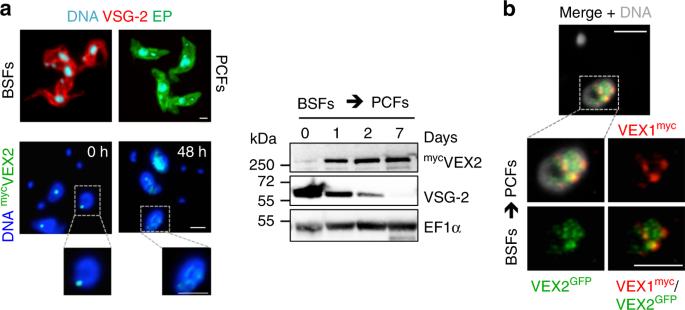Fig. 7 VEX-complex compartmentalisation is stage-specific.aImmunofluorescence and protein-blot analysis ofmycVEX2 localisation and expression, respectively, following differentiation of bloodstream forms (BSFs, 0 h) into procyclic forms (PCFs). As immunofluorescence control, the cells were stained for the major surface glycoprotein for each developmental stage; VSG in BSFs and EP-procyclin in PCFs. For protein blotting, EF1α was used as a loading-control.bGFPVEX2/VEX1myccolocalisation studies in 48 h differentiated BSFs. Inb, these images correspond to maximal 3D projections of 0.1 μm stacks. DNA was counter-stained with DAPI; scale bars 2 μm. Data representative of independent experiments. Source data are provided as a Source Data file Briefly, polyadenylated transcripts were enriched using poly-dT beads and reverse-transcribed before sequencing on a HiSeq platform (Illumina). Reads were mapped to a hybrid assembly consisting of the T. brucei 927 reference genome plus the bloodstream VSG -ESs [7] and metacyclic VSG- ESs [47] , [48] from the Lister 427 strain. Bowtie 2-mapping [49] was with the parameters --very-sensitive --no-discordant --phred33. Alignment files were manipulated with SAMtools [50] . Per-gene read counts were derived using the Artemis genome browser [63] , MapQ > 1 [18] . Read counts were normalised using edgeR [64] and differential expression was determined with classic edgeR. RPKM values were derived from normalised read counts in edgeR. Base pair resolution plots were generated using an in-house script. Statistical analysis All statistical analyses were performed using GraphPad Prism Software (version 7.0), except the transcriptomic analysis (described above). Detailed information regarding replicates, statistical tests and outputs can be found in Supplementary Data 1 , sheet 6. 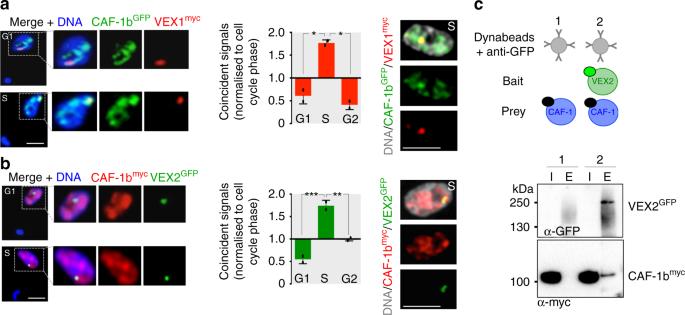Fig. 8 Colocalisation of CAF-1 and the VEX-complex during S phase.a,bImmunofluorescence-based colocalisation studies of VEX1myc/CAF-1bGFPand VEX2GFP/CAF-1bmyc. Representative images from G1 and S phase cells are shown. Nuclei (n≥ 70) were scored for CAF-1b puncta coincident with VEX1myc/VEX2GFPfoci. DNA was counter-stained with DAPI; scale bars, 2 μm. Error bars, SD; *p< 0.05; **p< 0.01; ***p< 0.001 (one-way ANOVA test). Values are averages from two independent biological replicates and are representative of independent experiments. The images on the right-hand side correspond to maximal 3D projections of 0.1 μm stacks.cCo-immunoprecipitation of VEX2GFP/CAF-1bmycfollowed by protein-blot analysis. Green circle, GFP; black circles, myc; I, input; E, elution. Source data are provided as a Source Data file 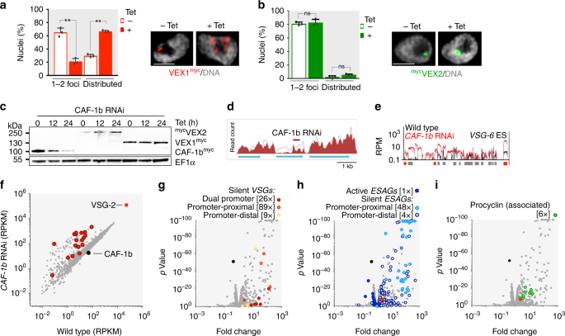Fig. 9 VEX-complex reassembly and inheritance requires CAF-1. VEX1myc(a), but notmycVEX2 (b), is distributed following tetracycline (Tet) induced CAF-1b knockdown (12 h), as assessed by immunofluorescence analysis. DNA was counter-stained with DAPI; scale bars, 2 μm. The images correspond to maximal 3D projections of 0.1 μm stacks. Error bars, SD; ns, not significant; **p< 0.01 (two-tailed paired Student’sttest). Values are averages from three independent biological replicates and are representative of independent experiments (the remaining cells displayed no detectable signal).cProtein-blot analysis of CAF-1bmyc,mycVEX2 and VEX1mycexpression following CAF-1b knockdown. EF1α was used as a loading-control.d–iRNA-seq analysis following CAF-1b knockdown (24 h).dTotal number of reads acrossCAF-1blocus in the parental population or followingCAF-1bRNAi.e–iValues are averages from two independent RNAi strains relative to wild-type controls. Paneleshows transcript abundance at the silentVSG-6ES. Red circles, promoters; red boxes,VSGs; grey boxes, other genes. RPKM/RPM, reads per (kilobase per) million (e–i). Panelsf–ihighlight different gene cohorts and numbers in square brackets indicate increase/decrease in total transcript abundance for each category; red square,VSG-2; black circle,CAF-1b. Promoter-proximalVSGsandESAGs(6, 7 and 10) are within 5 kbp of a promoter, distalVSGsare 46 +/−4 kbp from the promoter. Source data are provided as a Source Data file 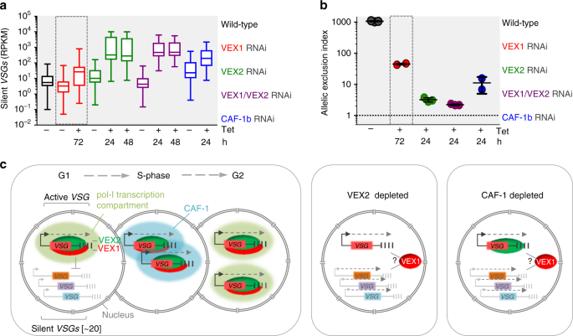Fig. 10 A model forVSGallelic exclusion by the VEX-complex.a,bComparative analysis ofVSG-transcripts from wild-typeT. bruceior following VEX1 (data from Glover et al., 2016; dashed boxes), VEX2, VEX1/VEX2 and CAF-1b knockdown (data from current study).aThe box-plot depicts the sum of silentVSGexpression; whiskers extend from the minimal to the maximal value, other details as in Fig.1a.bThe allelic exclusion index represents activeVSG-2expression divided by the expression of all other expression site associatedVSGscombined. Error bars, SD.cA model for heritable exclusion by the VEX-complex and CAF-1. Left-hand panel:VSG-ES transcription drives competition for a limited pool of the VEX-complex. Once associated with chromatin, the complex promotes transcription and transmits a silencing signal, excluding otherVSG-ESs, ultimately allowing only oneVSG-ES to recruit sufficient pol-I and to form a pol-I transcription compartment. CAF-1 dependent compartmentalisation of the complex provides allele-specific epigenetic inheritance. Middle and right-hand panels: VEX2 or CAF-1 depletion disrupts the VEX-complex associated transcription compartment and the silencing signal; it remains unclear how VEX1 interacts withVSG-ESs under these circumstances. Bent arrows and dashed arrows indicateVSG-ES promoters and transcription, respectively. Source data are provided as a Source Data file Resources and reagents Details of resources and reagents can be found in Supplementary Data 1 , sheet 7. All unique materials are available on request. Reporting summary Further information on research design is available in the Nature Research Reporting Summary linked to this article.